Nanodomain Ca2+of Ca2+channels detected by a tethered genetically encoded Ca2+sensor Coupling of excitation to secretion, contraction and transcription often relies on Ca 2+ computations within the nanodomain—a conceptual region extending tens of nanometers from the cytoplasmic mouth of Ca 2+ channels. Theory predicts that nanodomain Ca 2+ signals differ vastly from the slow submicromolar signals routinely observed in bulk cytoplasm. However, direct visualization of nanodomain Ca 2+ far exceeds optical resolution of spatially distributed Ca 2+ indicators. Here we couple an optical, genetically encoded Ca 2+ indicator (TN–XL) to the carboxy tail of Ca V 2.2 Ca 2+ channels, enabling near-field imaging of the nanodomain. Under total internal reflection fluorescence microscopy, we detect Ca 2+ responses indicative of large-amplitude pulses. Single-channel electrophysiology reveals a corresponding Ca 2+ influx of only 0.085 pA, and fluorescence resonance energy transfer measurements estimate TN–XL distance to the cytoplasmic mouth at ~55 Å. Altogether, these findings raise the possibility that Ca 2+ exits the channel through the analogue of molecular portals, mirroring the crystallographic images of side windows in voltage-gated K channels. Ca 2+ signals extend pervasively across the intracellular expanse of most cells; yet, these signals exhibit remarkable specificity in activating appropriate Ca 2+ -modulated targets. Understanding how this selectivity arises remains a foremost question in Ca 2+ biology [1] , [2] . One strategy is to co-localize at molecular dimensions Ca 2+ sources and targets. This co-localization is crucial to the local signalling of Ca 2+ channels to nearby Ca 2+ -regulated ion channels and enzymes [3] , [4] , [5] to neurotransmitter release [6] , as well as to excitation–contraction [7] and excitation–transcription coupling [8] , [9] . Intriguingly, co-localized sensors do not always respond preferentially to local Ca 2+ sources, but can require the far weaker input of remote Ca 2+ sources acting through a global Ca 2+ selectivity paradigm [10] . Critical to signalling near Ca 2+ sources is the nature of Ca 2+ signals within a few tens of nanometers of a Ca 2+ channel (nanodomain [11] ). Theoretical calculations [12] , [13] , [14] , [15] , [16] postulate that nanodomain signals comprise Ca 2+ pulses of equal and enormous amplitude (~100 μM), with each pulse synchronized to the millisecond stochastic openings of channels [10] , [12] . Beyond the nanodomain, [Ca 2+ ] rapidly dissipates with diffusion. Of note, predicted nanodomain [Ca 2+ ] amplitudes vary considerably with assumed parameters [17] , and elegant experimental estimates of local Ca 2+ signals [18] , [19] only indirectly probe the nanodomain itself. Thus, the critical magnitude of nanodomain Ca 2+ pulses ( Ca spike ) has eluded explicit empirical comment. This uncertainty bears on key issues, including how spatial Ca 2+ decoding occurs within the nanodomain [10] , [20] , [21] , [22] and the Ca 2+ channel number needed to trigger neurotransmitter vesicles [23] , [24] , [25] . Why have nanodomain Ca 2+ signals remained elusive? Although fluorescent Ca 2+ -sensitive chemical dyes have revealed much [26] , visualization of nanodomain signals via freely diffusible dye molecules far exceeds the resolution limit of far-field microscopic approaches [27] . In this regime, fluorescence from dye molecules outside the nanodomain will overshadow that from within [28] . Even when imaged with total internal reflection fluorescence (TIRF) microscopy [29] , [30] , [31] that illuminates a restricted TIRF volume within ~150 nm of the glass/cell membrane interface, freely diffusible dyes will still report Ca 2+ from a region several-fold larger than a Ca 2+ channel [32] . One approach is to affix a Ca 2+ indicator within the nanodomain, so as to support a form of near-field imaging [33] . The Ca 2+ -sensitive luminescent protein aequorin represents a traditional candidate [34] . Recombinant aequorins have long been targeted to various subcellular compartments by genetic means [35] , [36] , [37] but the limited-amplitude and consumptive nature of aequorin would challenge deployment in a channel nanodomain [34] . Recently, promising results have been obtained using a biarsenical chemical fluorescent Ca 2+ indicator (Calcium green FlAsH, CaGF) targeted to a tetracysteine tag implanted on Ca V 1.2 Ca 2+ channels [38] . CaGF features Ca 2+ affinity and kinetics ( K d , ~55 μM; off rate, 2 ms −1 ) well matched to the purported amplitudes and lifetimes of nanodomain Ca 2+ pulses. Indeed, CaGF was potentially responsive to nanodomain Ca 2+ fluctuations, but the observed fluorescence signals were highly heterogeneous, to an extent that precluded quantitative Ca 2+ estimation. This heterogeneity was attributable to the diminutive and variable open probability of Ca V 1.2 channels (~0.1–0.3%), despite constitutive pharmacological manipulation by a channel opener. Indeed, the possibility of a large fraction of electrically silent Ca V 1.2 channels fits with their unusually large ratio of gating charge to ionic current [39] . Also, although careful controls were performed for nonspecific labelling of other cysteine-rich sites in the cell by CaGF, such indiscriminate attachment would remain a generic concern for approaches involving chemical targeting of sensors. A third approach would be to employ genetically encoded Ca 2+ indicators (GECIs) as near-field sensors. GECIs allow genetic fusion of sensor to a Ca 2+ source, offering the greatest potential selectivity in positioning sensors. Among the most popular GECIs are CFP/YFP-FRET (fluorescence resonance energy transfer)-based molecules such as cameleons [40] , and GFP-intensity-based sensors like GCaMPs [41] . All these employ calmodulin (CaM) as their Ca 2+ sensor, and convert binding of the sensor's own Ca 2+ /CaM with a target peptide into altered optical readouts. When targeted to plasmalemma, cameleons often lose Ca 2+ sensitivity [42] , potentially via target peptide binding to elevated plasmalemmal CaM [43] . Accordingly, we here explore near-field imaging of nanodomain Ca 2+ using TN–XL, a GECI [44] based on the Ca 2+ sensor troponin C. TN–XL exploits Ca 2+ -driven conformational changes without a target peptide, thereby naturally resisting endogenous CaM interference [42] . Our specific approach is to fuse TN–XL to the carboxy terminus of the principle subunit of Ca V 2.2 Ca 2+ channels, chosen for high open probability [45] , relative absence of silent channels [46] , and abundant plasmalemmal expression [47] . To further improve the TN–XL signal-to-noise ratio at the surface membrane, we utilize TIRF microscopy to selectively illuminate only those Ca V 2.2/TN–XL channels near the surface, thereby attenuating background signal from imperfectly targeted intracellular channels. Finally, to account for the high Ca 2+ affinity and slow kinetics of GECIs [44] (off times, 100–900 ms for TN–XL) in the face of millisecond nanodomain Ca 2+ pulses, we quantify the kinetics of TN–XL readouts, which our previous work suggests can distinguish between differing Ca spike amplitudes [48] . These strategies allow us to resolve nanodomain Ca 2+ activity of Ca V 2.2 channels undergoing native gating, without pharmacological manipulation. Functional Ca V 2. 2/TN–XL fusions at the surface membrane Our strategy for probing nanodomain Ca 2+ signals ( Fig. 1 ) requires maintained Ca 2+ responsiveness of genetically encoded sensors situated at the plasmalemma, which is a foremost challenge. Accordingly, we examined whether troponin-based TN–XL could respond to Ca 2+ when targeted to this environment. As a baseline, Fig. 2a displays the properties of the well-studied, cytoplasmic form of TN–XL [44] . Confocal images of an exemplar HEK293 cell, acquired under CFP and FRET imaging modes, reveal the expected pan-cytoplasmic distribution. An epifluorescence CFP image of another cell also demonstrates this generalized expression, and switching to TIRF mode indicates no preferential TN–XL accumulation within the plasmalemmal footprint of this same cell. To gauge TN–XL responsiveness, we measured, under TIRF imaging, the single-cell CFP ( S C , respective excitation and emission wavelengths at 442 and 485 nm) and FRET fluorescence signals ( S F , excitation and emission at 442 and 545 nm), where the ratio of these signals ( R F/C = S F / S C ) furnishes the customary sensor readout of Ca 2+ ( Fig. 2b ). In particular, the ratio R F/C was first determined in resting cells with cytoplasmic Ca 2+ concentration (≤0.1 μM) well below the K d of the TN–XL [24] , thus yielding R min . To subsequently determine R max , Ca V 2.2 channels were co-expressed as conduits of Ca 2+ entry under whole-cell voltage clamp. To facilitate elevation of intracellular Ca 2+ , minimal internal Ca 2+ buffering (1 mM EGTA) with elevated 10 mM extracellular Ca 2+ was employed, such that repetitive step depolarizations (30 mV×500 ms pulses every 15 s) readily saturated R F/C at R max . Thus, the ratio of R max and R min reports sensor dynamic range. 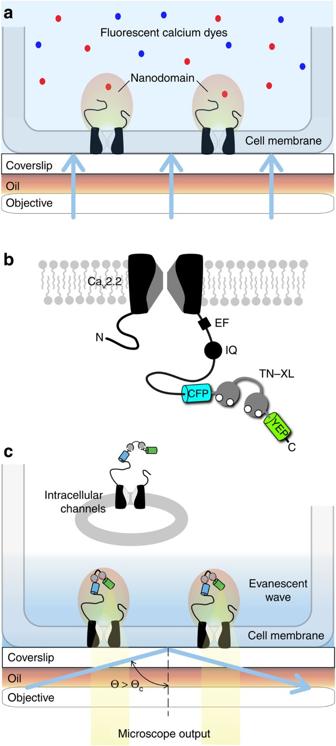Figure 1: Approach to resolving channel nanodomain Ca2+signals. (a) Conventional wide-field imaging using cytosolic chemical fluorescent dyes cannot resolve channel nanodomain Ca2+signals. Blue shading denotes region of fluorescence excitation, which extends throughout the cell under wide-field imaging. (b), Design of the genetically encoded Ca2+indicator TN–XL fused to the carboxy tail of theα1Bsubunit of a CaV2.2 channel, yielding CaV2.2/TN–XL. For orientation, structure-function elements involved in calmodulin regulation are denoted on carboxy terminus21: EF, EF-hand region; IQ, IQ-domain for apoCaM binding. CFP denotes enhanced CFP. YFP denotes circularly permuted citrine. (c), CaV2.2/TN–XL constructs act as a 'near-field' sensor of nanodomain Ca2+. TIRF imaging evanescent wave illuminates only CaV2.2/TN–XL channels within ~150 nm from the glass/cell membrane interface, as indicated by the blue-shaded region. This mode of excitation potentially excludes intracellular channels from consideration. When laser illumination angle Θ exceeds a critical angle ΘC, TIRF illumination occurs. Figure 1: Approach to resolving channel nanodomain Ca 2+ signals. ( a ) Conventional wide-field imaging using cytosolic chemical fluorescent dyes cannot resolve channel nanodomain Ca 2+ signals. Blue shading denotes region of fluorescence excitation, which extends throughout the cell under wide-field imaging. ( b ), Design of the genetically encoded Ca 2+ indicator TN–XL fused to the carboxy tail of the α 1B subunit of a Ca V 2.2 channel, yielding Ca V 2.2/TN–XL. For orientation, structure-function elements involved in calmodulin regulation are denoted on carboxy terminus [21] : EF, EF-hand region; IQ, IQ-domain for apoCaM binding. CFP denotes enhanced CFP. YFP denotes circularly permuted citrine. ( c ), Ca V 2.2/TN–XL constructs act as a 'near-field' sensor of nanodomain Ca 2+ . TIRF imaging evanescent wave illuminates only Ca V 2.2/TN–XL channels within ~150 nm from the glass/cell membrane interface, as indicated by the blue-shaded region. This mode of excitation potentially excludes intracellular channels from consideration. When laser illumination angle Θ exceeds a critical angle Θ C , TIRF illumination occurs. 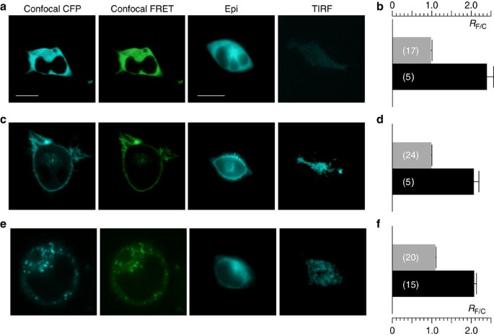Figure 2: CaV2.2/TN–XL fusion construct preserves function of sensor. (a) Behaviour of free TN–XL. Left to right: confocal (CFP filter), confocal (FRET filter), epi-fluorescence (CFP filter), and TIRF (CFP filter) images of HEK293 cells expressing cytoplasmic TN–XL. White scale bar, 10 μm. Bar at far left pertains to all confocal images. Bar at middle right pertains to all epifluorescence and TIRF images. (b) TN–XL ratio (RF/C=SF/SC) measured in resting cells (Rmin) (grey bar) and in cells under high Ca2+(Rmax) (black bar). Data shown as mean±s.e.m. with number of cells in parentheses. (c,d), Behaviour of TN–XL-Ras (membrane targeted TN–XL). Format as in (a,b), respectively. (e,f), Behaviour of 2/TN–XL (N-type channel fused to TN–XL). Format as in (a,b), respectively. Full size image Figure 2: Ca V 2.2/TN–XL fusion construct preserves function of sensor. ( a ) Behaviour of free TN–XL. Left to right: confocal (CFP filter), confocal (FRET filter), epi-fluorescence (CFP filter), and TIRF (CFP filter) images of HEK293 cells expressing cytoplasmic TN–XL. White scale bar, 10 μm. Bar at far left pertains to all confocal images. Bar at middle right pertains to all epifluorescence and TIRF images. ( b ) TN–XL ratio ( R F/C = S F / S C ) measured in resting cells ( R min ) (grey bar) and in cells under high Ca 2+ ( R max ) (black bar). Data shown as mean±s.e.m. with number of cells in parentheses. ( c , d ), Behaviour of TN–XL-Ras (membrane targeted TN–XL). Format as in ( a , b ), respectively. ( e , f ), Behaviour of 2/TN–XL (N-type channel fused to TN–XL). Format as in ( a , b ), respectively. Full size image By contrast, for TN–XL fused to the farnesylation motif of Ras (TN–XL-Ras), sensors are sharply localized to the surface membrane in confocal and epifluorescence images ( Fig. 2c ), and there is marked enrichment within the TIRF footprint. Importantly, the Ca 2+ dynamic range of TN–XL-Ras is nearly identical ( Fig. 2d ), despite residence within the plasmalemmal context. Yet more relevant are results for the Ca V 2.2/TN–XL fusions ( Fig. 2e ). Here constructs appear only partially localized to the surface membrane, consistent with typically imperfect trafficking of recombinant Ca 2+ channels to plasmalemma [49] . Still, there is substantial focalization of Ca V 2.2/TN–XL in the TIRF footprint, suggesting sufficient trafficking for nanodomain experiments ( Fig. 1c ). Critically, sensor dynamic range is spared when juxtaposed near Ca V 2.2 channels ( Fig. 2f ). A second concern is the preservation of Ca V 2.2 channel function upon fusion to TN–XL. Reassuringly, Ca 2+ currents appeared nearly identical in Ca V 2.2/TN–XL ( Fig. 3a , black) and Ca V 2.2 (grey) channels. In fact, fusing TN–XL to Ca V 2.2 enhances opening, as seen from hyperpolarization of tail-activation curves determined with 10-mM extracellular Ca 2+ as charge carrier ( Fig. 3b ). Even at the single-channel level, Ca V 2.2/TN–XL fusions exhibited robust electrophysiological function, as illustrated by the exemplar single-channel current trace shown at high-gain magnification ( Fig. 3c , noisy trace). We used 90 mM Ba 2+ as a charge carrier to enhance resolution of elementary events, and evoked currents via ramp depolarization to readily resolve the open-channel conduction profile (downwardly convex grey relation). Multiple single-channel sweeps ( Fig. 3d ), displayed at lower-gain magnification, confirm the overall reproducibility and excellent resolution of elementary events under this protocol. Accordingly, numerous sweeps from multiple patches specify a highly reliable ensemble average current ( Fig. 3c , red curve), closely similar to that of Ca V 2.2 channels without sensor fusion [45] . Taking the ratio of the ensemble average current with the open-channel conduction profile ( Fig. 3c , red and convex grey curves) yields a plot of open probability P O versus voltage V ( Fig. 3e , gray relation). This plot matches impressively with whole-cell activation (reproduced as open circles), after shifting along the voltage axis to account for contrasting surface-charge effects of single-channel versus whole-cell solutions. As with studies of Ca V 2.2 (ref. 45 ), the Ca V 2.2/TN–XL fusion exhibits a substantial P O of 0.69 at 30 mV ( Fig. 3e , red arrows), a feature advantageous for probing nanodomain Ca 2+ . 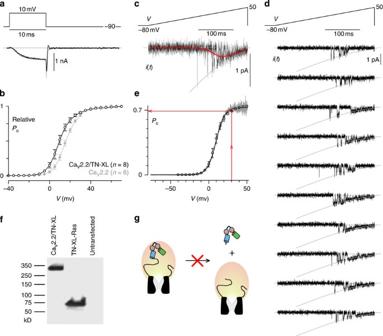Figure 3: CaV2.2/TN–XL fusion construct preserves function of channel. (a) Exemplar whole-cell currents of HEK293 cells expressing 2 channels (grey) or 2/TN–XL channels (black), using 10 mM Ca2+as charge carrier, and 10 mM EGTA intracellular Ca2+buffering. (b), Whole-cell tail-activation curves of 2 (grey) and 2/TN–XL (black), obtained from records as in (a). Data shown as mean±s.e.m. with number of cells in parentheses. (c), Single-channel analysis of 2/TN–XL. Top, On-cell ramp-voltage waveform delivered every 5–15 s. Bottom, exemplar single-channel sweep shown at high-gain magnification (100–200 per patch). 90 mM Ba2+as charge carrier; 2 kHz low-pass filtering. Leak-subtracted traces were averaged, yielding redI-Vcurve. Unitary current relation (convex grey curve) was fitted to the open-channel current level using GHK equation10. (d), Multiple exemplar single-channel sweeps from another patch, shown at lower-gain magnification to impart a sense of the overall reproducibility and excellent resolution of elementary events. Format as inc. (e), Single-channelPO–Vrelation (grey, with fit in black, average ofn=4 patches), determined by dividingI-Vcurve (c, red trace) by unitary current relation (c, grey, GHK fit).PO–Vcurve was calibrated in voltage by aligning the single-channel activation curve with the whole-cell curve reproduced from (b) (open circles). From calibratedPO–Vcurve, thePoat 30 mV is 0.69. (f) Immunoblots of HEK293 cell lysates probed with anti-GFP antibody; (left) 2/TN–XL at ~320 kD; (middle) TN–XL-Ras at ~71 kD; (right) control (untransfected) cells for reference. (g) Lack of lower molecular-weight species in leftmost lane of (f) excludes proteolysis of sensor from channel. Figure 3: Ca V 2.2/TN–XL fusion construct preserves function of channel. ( a ) Exemplar whole-cell currents of HEK293 cells expressing 2 channels (grey) or 2/TN–XL channels (black), using 10 mM Ca 2+ as charge carrier, and 10 mM EGTA intracellular Ca 2+ buffering. ( b ), Whole-cell tail-activation curves of 2 (grey) and 2/TN–XL (black), obtained from records as in ( a ). Data shown as mean±s.e.m. with number of cells in parentheses. ( c ), Single-channel analysis of 2/TN–XL. Top, On-cell ramp-voltage waveform delivered every 5–15 s. Bottom, exemplar single-channel sweep shown at high-gain magnification (100–200 per patch). 90 mM Ba 2+ as charge carrier; 2 kHz low-pass filtering. Leak-subtracted traces were averaged, yielding red I-V curve. Unitary current relation (convex grey curve) was fitted to the open-channel current level using GHK equation [10] . ( d ), Multiple exemplar single-channel sweeps from another patch, shown at lower-gain magnification to impart a sense of the overall reproducibility and excellent resolution of elementary events. Format as in c . ( e ), Single-channel P O – V relation (grey, with fit in black, average of n =4 patches), determined by dividing I - V curve ( c , red trace) by unitary current relation ( c , grey, GHK fit). P O – V curve was calibrated in voltage by aligning the single-channel activation curve with the whole-cell curve reproduced from ( b ) (open circles). From calibrated P O – V curve, the P o at 30 mV is 0.69. ( f ) Immunoblots of HEK293 cell lysates probed with anti-GFP antibody; (left) 2/TN–XL at ~320 kD; (middle) TN–XL-Ras at ~71 kD; (right) control (untransfected) cells for reference. ( g ) Lack of lower molecular-weight species in leftmost lane of ( f ) excludes proteolysis of sensor from channel. Full size image A final prerequisite is that Ca V 2.2/TN–XL fusions resist proteolysis. Accordingly, we utilized anti-GFP antibody to perform western immunoblots from cells expressing this construct ( Fig. 3f , left lane). The other lanes correspond to cells expressing TN–XL-Ras (~71 kD), as well as untransfected cells (no signal). The absence of signal beneath the full-length ~320 kD band ( Fig. 3f , left lane) substantiates maintained TN–XL fusion to channels ( Fig. 3g ). Calibration of TN–XL fused to Ca V 2.2. channels We next addressed more precise sensor calibration, to facilitate quantitative inferences about nanodomain Ca 2+ . Both kinetic and steady-state characterization would be ideal, given the millisecond kinetics of Ca 2+ pulses within channel nanodomains, coupled with the comparatively slow response of free TN–XL (off rates of 1/150 to 1/850 1/ms [44] ). Accordingly, we devised a state-mechanism approximation of sensor performance, a 'forward transform' that maps rapid Ca 2+ transient inputs onto slower sensor outputs, as previously established for an older variant of TN–XL (TN-L15), freely expressed in myocytes [48] . Here we pursued an analogous approach, but attuned to Ca V 2.2/TN–XL constructs resident within the TIRF volume and driven by high-amplitude dynamic Ca 2+ inputs pertinent to channel nanodomains. To produce such inputs, we activated ultra-large Ca V 2.2 Ca 2+ currents ( Fig. 4a ) in HEK293 cells, featuring minimal exogenous intracellular Ca 2+ buffering (1 mM EGTA); this configuration intentionally produced enormous spatial gradients of intracellular Ca 2+ ( Fig. 4b , inset), far exceeding that usually encountered. To estimate these gradients, we simultaneously monitored aggregate Ca 2+ concentration ( Fig. 4b , noisy dark trace), as deduced by imaging the entire cell for signals emanating from 10 μM of the rapid chemical fluorescent Ca 2+ indicator Fluo 4FF. The measured Ca 2+ influx ( Fig. 4a ) and aggregate [Ca 2+ ] signals were then used to explicitly constrain a radially symmetric Ca 2+ diffusion mechanism, whose estimates of Ca 2+ concentration, in differing cellular regions, are shown as red traces in Fig. 4b ( Supplementary Fig. S1; Supplementary Methods ). The estimated aggregate [Ca 2+ ] concentration ( Fig. 4b , lower red trace) closely approximates its measured analogue (dark noisy trace), and the estimated [Ca 2+ ] at the surface membrane (upper red trace) peaks at ~80 μM and later converges to the aggregate [Ca 2+ ] (~20–25 μM). This estimate of submembranous [Ca 2+ ] was reproducible in multiple cells exhibiting like Ca 2+ influx, and was thereby taken as the relevant Ca 2+ input in parallel experiments performed with Ca V 2.2/TN–XL fusion constructs, under TIRF imaging. The green trace in Fig. 4c displays the corresponding sensor output from GECIs in the submembranous TIRF volume, averaged from multiple cells exhibiting Ca 2+ influx matching that in Fig. 4a . The steady-state plateau of the response ( Fig. 4c , grey dashed line at R F/C =1.78), at a near steady Ca 2+ concentration of ~20–25 μM, enabled us to calculate ~17.3 μM as the half-response point of the steady-state response curve for Ca V 2.2/TN–XL constructs in the TIRF volume ( Supplementary Methods ). This differs from the 2.5 μM half-response point for free TN–XL [44] , consistent with previous observations that sensor performance can change with cellular/molecular environment [38] , [42] . Accordingly, steady-state response data for free TN–XL [44] were shifted along the [Ca 2+ ] axis by ×16.3/2.5 to provide an appropriate steady-state profile for Ca V 2.2/TN–XL constructs ( Fig. 4d , green symbols). In all, these steady-state data and the dynamic sensor response ( Fig. 4c , green trace) to a specified submembranous Ca 2+ input ( Fig. 4b , upper red trace) furnished the constraints required to deduce a forward transform for Ca V 2.2/TN–XL. 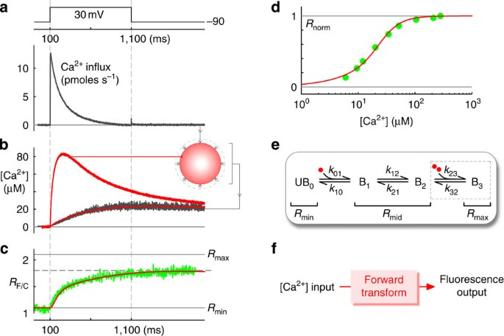Figure 4: Calibration of CaV2.2/TN–XL fusion construct. (a) High-amplitude Ca2+influx into HEK293 cell expressing CaV2.2 channels, observed with 10 mM external Ca2+and minimal internal Ca2+buffering of 1 mM EGTA. (b) Simultaneous [Ca2+] measurement (dark trace) deduced from 10 μM Fluo-4FF Ca2+-indicator fluorescence from entirety of same cell (514 nm excitation, 545 nm emission). Ca2+determination rendered ratiometric by inclusion of 2.5 μM red Alexa 568 dye (514 nm excitation, 580 nm long-pass emission). Inset, cartoon of spatial Ca2+gradients in this cell. Red traces, projected [Ca2+] waveforms from Ca2+diffusion mechanism constrained by Ca2+input in (a) and aggregate [Ca2+] (dark trace): lower red trace, aggregate [Ca2+]; upper red trace, submembranous [Ca2+]. (c), Average FRET-ratio (RF/C) response of CaV2.2/TN–XL channels in TIRF volume (green trace); same protocol as in (a,b). Red trace, output of TN–XL forward transform in (e), when driven by submembranous [Ca2+] input (b, upper red trace). (d) Normalized steady-state FRET-ratio response (Rnorm=(RF/C−Rmin)/(Rmax−Rmin) of CaV2.2/TN–XL to [Ca2+] (experimental green symbols). Red trace, steady-state output of TN–XL forward transform in (e) when driven by differing fixed [Ca2+]. (e) State-diagram representation of CaV2.2/TN–XL. Red circles, Ca2+ions. UB, conformation with no calcium bound. B, various conformations with calcium bound. (f) System of states and corresponding fluorescence/FRET properties constitutes a forward transform that predicts TN–XL sensor outputs as a function of time-varying Ca2+inputs.1) Figure 4: Calibration of Ca V 2.2/TN–XL fusion construct. ( a ) High-amplitude Ca 2+ influx into HEK293 cell expressing Ca V 2.2 channels, observed with 10 mM external Ca 2+ and minimal internal Ca 2+ buffering of 1 mM EGTA. ( b ) Simultaneous [Ca 2+ ] measurement (dark trace) deduced from 10 μM Fluo-4FF Ca 2+ -indicator fluorescence from entirety of same cell (514 nm excitation, 545 nm emission). Ca 2+ determination rendered ratiometric by inclusion of 2.5 μM red Alexa 568 dye (514 nm excitation, 580 nm long-pass emission). Inset, cartoon of spatial Ca 2+ gradients in this cell. Red traces, projected [Ca 2+ ] waveforms from Ca 2+ diffusion mechanism constrained by Ca 2+ input in ( a ) and aggregate [Ca 2+ ] (dark trace): lower red trace, aggregate [Ca 2+ ]; upper red trace, submembranous [Ca 2+ ]. ( c ), Average FRET-ratio ( R F/C ) response of Ca V 2.2/TN–XL channels in TIRF volume (green trace); same protocol as in ( a , b ). Red trace, output of TN–XL forward transform in ( e ), when driven by submembranous [Ca 2+ ] input ( b , upper red trace). ( d ) Normalized steady-state FRET-ratio response ( R norm =( R F/C − R min )/( R max − R min ) of Ca V 2.2/TN–XL to [Ca 2+ ] (experimental green symbols). Red trace, steady-state output of TN–XL forward transform in ( e ) when driven by differing fixed [Ca 2+ ]. ( e ) State-diagram representation of Ca V 2.2/TN–XL. Red circles, Ca 2+ ions. UB, conformation with no calcium bound. B, various conformations with calcium bound. ( f ) System of states and corresponding fluorescence/FRET properties constitutes a forward transform that predicts TN–XL sensor outputs as a function of time-varying Ca 2+ inputs.1) Full size image Fig. 4e displays the corresponding state-diagram approximation of Ca V 2.2/TN–XL responsiveness to Ca 2+ , based on a mechanism for an older troponin-based GECI [48] (TN-L15). State UB 0 ('unbound') represents the Ca 2+ -free conformation of the sensor, characterized by a lower FRET-ratio output of R min . On binding of a single Ca 2+ to the N-lobe of troponin, the sensor adopts one of two alternate 'bound' conformations (B 1 or B 2 ), both featuring the same elevated FRET-ratio output of R mid . The arrangement, thus far, is identical to that previously established for TN-L15 (ref. 48 ). The improved performance of TN–XL arises, via engineering the C-lobe of troponin, to dynamically bind and unbind two signalling Ca 2+ ions, thereby driving a further conformational change of the sensor [44] . To account for this feature, we allowed two additional Ca 2+ ions to bind and induce a third bound state [50] , [51] (B 3 , dashed box), exhibiting the highest FRET-ratio output of R max . Numerical simulations of this scheme ( Supplementary Methods ), coupled with error minimization via parameter variation, yielded impressive fits to the target constraints above ( Fig. 4c,d , red curves), using the sensor parameter estimates in Table 1 . Accordingly, these parameters and the scheme in Fig. 4e furnish a steady-state and dynamic representation of Ca V 2.2/TN–XL responsiveness to Ca 2+ , a 'forward transform' ( Fig. 4f ) that is potentially appropriate for making inferences about channel nanodomain Ca 2+ fluctuations. Table 1 Full size table Ca V 2.2/TN–XL sensors respond to nanodomain Ca 2+ signals This transform could only be utilized, however, if a substantial fraction of Ca V 2.2/TN–XL sensors respond to channel nanodomain Ca 2+ signals, as specifically produced by individual channels fluxing Ca 2+ into their own nanodomain. Thus far, we had only demonstrated that Ca V 2.2/TN–XL sensors in the TIRF volume respond well to a generalized increase in submembranous [Ca 2+ ], but this would occur whether the majority of channel-sensor fusion constructs are properly trafficked to the surface membrane, or still plentiful in submembranous vesicles within the TIRF volume. To address this issue, we again undertook simultaneous recordings of whole-cell Ca 2+ current and TIRF imaging of Ca V 2.2/TN–XL sensors, but here with high intracellular Ca 2+ buffering present to restrict Ca 2+ elevations to the nanodomain of active channels that flux Ca 2+ . Specifically, we dialysed cells with 10 mM EGTA, yielding a Ca 2+ nanodomain radius of ~40 nm (ref. 13 ) ( Fig. 5 , top cartoon), only twofold larger than electron micrographic estimates of Ca 2+ channel diameters [32] . Additionally, we only investigated cells with modest Ca 2+ currents (~1 nA with 10 mM Ca 2+ as charge carrier) and little Ca 2+ -dependent inactivation [21] (CDI), so as to exclude Ca 2+ buffer depletion. Fig. 5a summarizes the results of an exemplar cell satisfying this criterion, with the displayed data evoked by a single voltage pulse. Clearly present is a transient decrease in CFP fluorescence ( S C , cyan trace), accompanied by a corresponding phasic elevation of the FRET ratio R F/C (green trace). Exponential fits (solid black curves) revealed dominant rise and fall times of 880 and 2,000 ms for S C , and 880 and 400 ms for R F/C . Both the return of TN–XL waveforms towards baseline, and the modest CDI of channels under elevated Ca 2+ buffering [21] ( Fig. 5a compared with Fig. 4a ), argue against unintended depletion of Ca 2+ buffer. Accordingly, these results suggest responsiveness of Ca V 2.2/TN–XL sensors to genuine channel nanodomain Ca 2+ signals. By contrast to the exemplar, about half the cells with currents of this magnitude and limited CDI exhibited no appreciable change of TN–XL readouts, presumably due to poor trafficking of active channels. Such cells were excluded from further analysis. 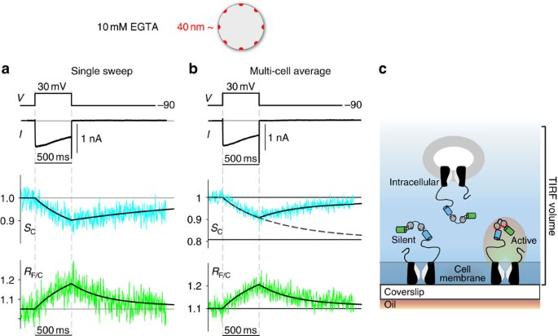Figure 5: CaV2.2/TN–XL sensors respond to channel nanodomain Ca2+signals. Top cartoon, Ca2+nanodomains under elevated Ca2+buffering, where Ca2+elevation is restricted to nanodomains, each affiliated with individual channel. 40 nm nanodomain calculated with equation (1),f=1 (classical assumption), unitary currenti=0.085 pA, and conservatively requiring [Ca2+] ~60 nM (the approximate resting physiological Ca2+concentration). (a) Simultaneous records of whole-cell current (top) and TIRF fluorescence signals (middle and bottom) from HEK293 cell expressing 2/TN–XL, using 10 mM external Ca2+and 10 mM internal EGTA Ca2+buffering. Shown are data from a single trial, evoked by the first step depolarization in the cell. Top, voltage and current waveforms, with moderately sized current chosen to minimize buffer consumption. Middle, corresponding CFP fluorescence signal after normalization to baseline level (SC, noisy trace). Black curve, approximate exponential fits (initial phase: 200 ms (10%), 880 ms (90%); recovery phase: 2,000 ms (100%)). Vertical ticks, 0.1 increment. Bottom, corresponding FRET-ratio signal (RF/C, noisy trace). Black curve, approximate exponential fits (initial phase: 200 ms (10%), 880 ms (90%); recovery phase: 400 msec (70%), 2,000 ms (30%)). Vertical ticks, 0.1 increment. (b) Average 2/TN–XL responses to nanodomain Ca2+signals, as isolated with 10 mM internal EGTA Ca2+buffering. Protocol and format as in (a).n=4 cells, with records taken from the first-step depolarization delivered in cells. CDI sometimes increased with repeated depolarizations, reflecting buffer depletion with attendant slowing ofRF/Cwaveform decay. Cells exhibiting peak currents ≤ 500 pA were not considered, as these cells demonstrated negligibleRF/Ctransients, presumably reflecting insufficient trafficking of active channels. Solid-black-curve exponential fits were similar, withSCexponential fit (initial phase: 200 ms (10%), 880 ms (90%); recovery phase: 500 ms (80%), 2,500 ms (20%)), andRF/Cfit (initial phase: 200 ms (10%), 880 ms (90%); recovery phase: 400 msec (70%), 2,000 ms (30%)). Dashed black curve, continuation of initial phaseSCexponential fit, which asymptotes at lower horizontal black line in middle. (c) Schematic of various classes of 2/TN–XL species in TIRF volume. Blue shading indicates region of excitation by evanscent wave in TIRF volume. Figure 5: Ca V 2.2/TN–XL sensors respond to channel nanodomain Ca 2+ signals. Top cartoon, Ca 2+ nanodomains under elevated Ca 2+ buffering, where Ca 2+ elevation is restricted to nanodomains, each affiliated with individual channel. 40 nm nanodomain calculated with equation (1), f =1 (classical assumption), unitary current i =0.085 pA, and conservatively requiring [Ca 2+ ] ~60 nM (the approximate resting physiological Ca 2+ concentration). ( a ) Simultaneous records of whole-cell current (top) and TIRF fluorescence signals (middle and bottom) from HEK293 cell expressing 2/TN–XL, using 10 mM external Ca 2+ and 10 mM internal EGTA Ca 2+ buffering. Shown are data from a single trial, evoked by the first step depolarization in the cell. Top, voltage and current waveforms, with moderately sized current chosen to minimize buffer consumption. Middle, corresponding CFP fluorescence signal after normalization to baseline level ( S C , noisy trace). Black curve, approximate exponential fits (initial phase: 200 ms (10%), 880 ms (90%); recovery phase: 2,000 ms (100%)). Vertical ticks, 0.1 increment. Bottom, corresponding FRET-ratio signal ( R F/C , noisy trace). Black curve, approximate exponential fits (initial phase: 200 ms (10%), 880 ms (90%); recovery phase: 400 msec (70%), 2,000 ms (30%)). Vertical ticks, 0.1 increment. ( b ) Average 2/TN–XL responses to nanodomain Ca 2+ signals, as isolated with 10 mM internal EGTA Ca 2+ buffering. Protocol and format as in ( a ). n =4 cells, with records taken from the first-step depolarization delivered in cells. CDI sometimes increased with repeated depolarizations, reflecting buffer depletion with attendant slowing of R F/C waveform decay. Cells exhibiting peak currents ≤ 500 pA were not considered, as these cells demonstrated negligible R F/C transients, presumably reflecting insufficient trafficking of active channels. Solid-black-curve exponential fits were similar, with S C exponential fit (initial phase: 200 ms (10%), 880 ms (90%); recovery phase: 500 ms (80%), 2,500 ms (20%)), and R F/C fit (initial phase: 200 ms (10%), 880 ms (90%); recovery phase: 400 msec (70%), 2,000 ms (30%)). Dashed black curve, continuation of initial phase S C exponential fit, which asymptotes at lower horizontal black line in middle. ( c ) Schematic of various classes of 2/TN–XL species in TIRF volume. Blue shading indicates region of excitation by evanscent wave in TIRF volume. Full size image Forward transform estimates of nanodomain Ca 2+ amplitudes As a prelude to more rigorous assessment of Ca V 2.2/TN–XL responses to nanodomain signals, we averaged signals from multiple responsive cells dialysed with 10 mM EGTA. The mean responses ( Fig. 5b ) were similar to those of the exemplar, with nearly identical characteristic time constants. This reproducibility encouraged us to quantitatively scrutinize these averaged waveforms. In particular, although the robust responses observed here under elevated Ca 2+ buffering do indicate an appreciable fraction of active channels within the TIRF volume ( Fig. 5c , active), the data do not exclude the possibility of a still substantial fraction of channels that are present in the plasmalemma but fail to open ( Fig. 5c , silent), or resident within submembranous vesicles within the TIRF volume ( Fig. 5c , intracellular). Such silent and/or intracellular channels would contribute static background fluorescence that could complicate quantitative interpretation. An indication of this scenario comes from exponential extrapolation of the S C waveform decline ( Fig. 5b , dashed curve), which asymptotes in the range of ~0.8. By contrast, under the assumption that all channels are active, simulations of the forward transform in Fig 4e,f indicate that, over a large range of plausible nanodomain Ca 2+ pulse amplitudes (≥35 μM), S C waveforms would asymptote near Ca 2+ -saturating levels of ~0.5 ( Supplementary Fig. S2 ; Supplementary Methods ), as specified by the experimentally determined 1/ α 0 value (defined in Table 1 ). Hence, the experimentally deduced asymptote of ~0.8 ( Fig. 5b ) suggests that ~40% of Ca V 2.2/TN–XL channels are active within the TIRF volume, whereas ~60% of channels are intracellular or silent. Cognizant of this configuration, we correct S C and R F/C waveforms to reflect only active channels, simply by subtracting ~60% of the baseline amplitude of CFP ( S C ) and FRET ( S F ) signals, and taking a ratio of these subtracted signals to obtain a corrected R F/C . Fig. 6a shows the corrected signals ( ), averaged over multiple cells. These waveforms were then suitable for making inferences about nanodomain Ca 2+ . 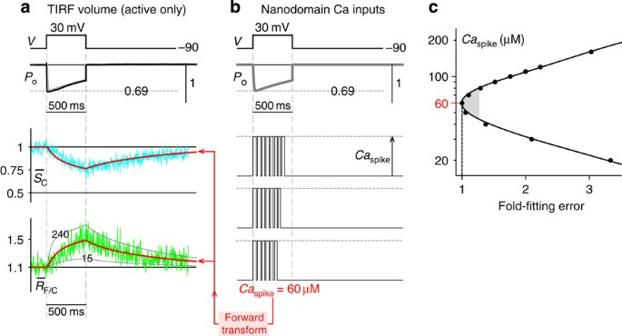Figure 6: Estimates of nanodomain Ca2+amplitude from CaV2.2/TN–XL responses. (a) Average CaV2.2/TN–XL responses to nanodomain Ca2+signals, corrected to reflect signal of active channels alone. Top, black trace plots average whole-current, rescaled to open probabilityPOby normalizing peak current during 30-mV pulse to 0.69. Grey trace, exponential fit toPOwaveform. Middle, cyan trace plots averageC, corrected CFP signal. Red trace, forward transform prediction of experimentalCusingCaspike=60 μM. Bottom, Green trace plots average, corrected FRET-ratio signal. Red trace, forward transform prediction of experimentalusingCaspike=60 μM. Grey traces, transform prediction withCaspikeas labelled. (b), Nanodomain Ca2+signals input to forward transform for prediction of CaV2.2/TN–XL responses in (a). Top,POwaveform reproduced from (a). Middle, Schematic of stochastic Ca2+pulses in nanodomain. Bottom, forward transform box with parameters inTable 1. (c)Caspikeestimation criteria. PresumedCaspikevalues plotted versus fold-fitting error (sum of squared deviations between fit and data, normalized to sum withCaspike=60 μM). Cusp of plot denotesCaspike=60 μM as best fit. Shaded zone specifies approximate confidence region, where fits yield errors within 25% of minimum. Figure 6: Estimates of nanodomain Ca 2+ amplitude from Ca V 2.2/TN–XL responses. ( a ) Average Ca V 2.2/TN–XL responses to nanodomain Ca 2+ signals, corrected to reflect signal of active channels alone. Top, black trace plots average whole-current, rescaled to open probability P O by normalizing peak current during 30-mV pulse to 0.69. Grey trace, exponential fit to P O waveform. Middle, cyan trace plots average C , corrected CFP signal. Red trace, forward transform prediction of experimental C using Ca spike =60 μM. Bottom, Green trace plots average , corrected FRET-ratio signal. Red trace, forward transform prediction of experimental using Ca spike =60 μM. Grey traces, transform prediction with Ca spike as labelled. ( b ), Nanodomain Ca 2+ signals input to forward transform for prediction of Ca V 2.2/TN–XL responses in ( a ). Top, P O waveform reproduced from ( a ). Middle, Schematic of stochastic Ca 2+ pulses in nanodomain. Bottom, forward transform box with parameters in Table 1 . ( c ) Ca spike estimation criteria. Presumed Ca spike values plotted versus fold-fitting error (sum of squared deviations between fit and data, normalized to sum with Ca spike =60 μM). Cusp of plot denotes Ca spike =60 μM as best fit. Shaded zone specifies approximate confidence region, where fits yield errors within 25% of minimum. Full size image That nanodomain Ca 2+ signals take the form of equi-amplitude Ca 2+ pulses, synchronized to the millisecond opening of channels, is widely accepted [10] , [12] (cartoon, Fig. 6b ); however, the critical amplitude of such pulses ( Ca spike ) has only been inferred via simulations of Ca 2+ diffusion [12] , [13] , [14] , [15] , [16] . To estimate Ca spike empirically, we analysed the corrected Ca V 2.2/TN–XL responses ( Fig. 6a ), using the forward transform in Fig. 4e,f . The experimental waveforms might initially appear difficult to conceptualize, as each TN–XL sees a different stochastic record of Ca 2+ pulses driven by single-channel openings. However, because the response of each TN–XL is slow ( Table 1 ; compare Fig. 4b,c ), relative to the millisecond duration of individual Ca 2+ spikes, we can adopt a previously established kinetic simplification [10] that permits the Ca 2+ -driven forward reaction rates in Fig. 4e to be treated, not as stochastic entities that fluctuate with each Ca 2+ pulse, but as smoothly changing entities and . Importantly, these entities are to the first order equal for all active Ca V 2.2/TN–XL sensors, such that the collective output from multiple sensors, as displayed in Fig. 6a , would approximate that for any individual sensor on average. Thus, using our forward transform ( Fig. 4e,f ) to predict experimental waveforms becomes simple. Single-channel data ( Fig. 3e ) permit average whole-cell currents ( Fig. 5b ) to be rescaled as an open probability P O waveform ( Fig. 6a,b ); this P O drives straightforward numerical integration of the differential equations corresponding to the transform in Fig. 4e , and this integration yields predictions of experimental waveforms, with the magnitude of Ca spike , being the only unknown ( Supplementary Methods ). Whereas presumed Ca spike values of 15 or 240 μM yield predicted trajectories ( Fig. 6a , grey smooth curves) that are patently inconsistent with the experimental curve, Ca spike =60 μM produces an impressive fit to data (smooth red curves). Indeed, error analysis ( Fig. 6c ) confirms 60 μM as a best estimate of Ca spike . As a conservative lower limit, we performed transform analysis on uncorrected waveforms ( Fig. 5b ), yielding a still-large estimated Ca spike ~15 μM ( Supplementary Fig. S3 ; Supplementary Methods ). Fits to uncorrected data were notably inferior, further prompting us to favour Ca spike estimates from the background-corrected data in Fig. 6a . For these data, the shading in Fig. 6c encompasses fits with errors similar to the minimum, yielding an approximate Ca spike range of 45–80 μM. This estimate, combined with determination of the underlying single-channel current amplitude, can potentially furnish valuable insight into Ca 2+ diffusion properties within the nanodomain itself ( Fig. 7 ). 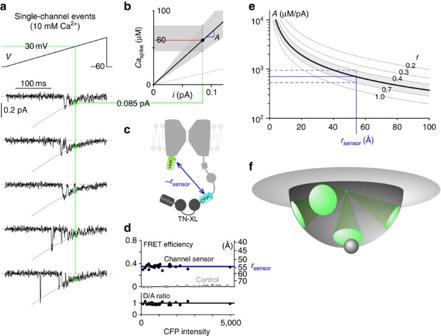Figure 7: Potential fenestrated Ca2+egress within CaV2.2 channel nanodomain. (a) On-cell single-channel ramp experiments, with 10 mM Ca2+as charge carrier to accord with whole-cell experiments; 700-Hz low-pass filtering. Voltages adjusted to align single-channel activation with whole-cell activation curves. Exemplars from single patch, with openings to GHK relation (grey curve). Unitary currentiat 30 mV (green circles), 0.085 pA in 5 patches. (b) Gain factorA, slope ofCaspikeversusirelation. Shading, various estimates ofAover confidence range ofCaspike. Sloped dashed line, lower-limit estimate ofAusing uncorrected data. (c) Schematic, FRET construct to estimatersensor. Substituting circularly permuted amber for circularly permuted Citrine of TN–XL maintains sensor-channel configuration. (d) Estimatingrsensorvia FRET. Each black symbol, individual HEK293 cell expressing construct in (c). Two outputs for each such cell obtained via 33-FRET analysis54of fluorescence images: FRET efficiency and ratio of donor (CFP) to acceptor (YFP) molecules (D/A ratio), both plotted versus CFP intensity (construct expression level). Data from cells exhibiting D/A ratio ~1 (as expected fromc) are displayed and analysed (bottom subpanel, black line at unity). Invariant FRET efficiency with increasing CFP intensity (top subpanel) excludes spurious FRET, facilitating interpretation of FRET efficiency (~0.35, blue line, top subpanel, left axis) as indicative ofrsensor~55 Å (top subpanel, right axis). Grey symbols, control cells expressing YFP and CFP separately, yielding efficiencies ~0. (e)Aversus sensor distance from channel mouth (rsensor), calculated with Neher-Stern equation (equation (1)), using parameters13,60DCa=0.4 μm2ms−1andkBon=10−3μM−1ms−1for EGTA. Grey curves, plots withfvalues as labelled. MappingAfrom (b) withrsensorfrom (d) yieldsf~0.53 (black curve) and range (0.4-0.7, shading). (f) Schematic, idealized fenestrated Ca2+egress from inner channel mouth. Green cones, permissive radial diffusion paths from source (green dot), summing tof~0.53. Target molecule (grey ball) within/near portal enjoys preferential signalling. Figure 7: Potential fenestrated Ca 2+ egress within Ca V 2.2 channel nanodomain. ( a ) On-cell single-channel ramp experiments, with 10 mM Ca 2+ as charge carrier to accord with whole-cell experiments; 700-Hz low-pass filtering. Voltages adjusted to align single-channel activation with whole-cell activation curves. Exemplars from single patch, with openings to GHK relation (grey curve). Unitary current i at 30 mV (green circles), 0.085 pA in 5 patches. ( b ) Gain factor A , slope of Ca spike versus i relation. Shading, various estimates of A over confidence range of Ca spike . Sloped dashed line, lower-limit estimate of A using uncorrected data. ( c ) Schematic, FRET construct to estimate r sensor . Substituting circularly permuted amber for circularly permuted Citrine of TN–XL maintains sensor-channel configuration. ( d ) Estimating r sensor via FRET. Each black symbol, individual HEK293 cell expressing construct in ( c ). Two outputs for each such cell obtained via 3 3 -FRET analysis [54] of fluorescence images: FRET efficiency and ratio of donor (CFP) to acceptor (YFP) molecules (D/A ratio), both plotted versus CFP intensity ( construct expression level). Data from cells exhibiting D/A ratio ~1 (as expected from c ) are displayed and analysed (bottom subpanel, black line at unity). Invariant FRET efficiency with increasing CFP intensity (top subpanel) excludes spurious FRET, facilitating interpretation of FRET efficiency (~0.35, blue line, top subpanel, left axis) as indicative of r sensor ~55 Å (top subpanel, right axis). Grey symbols, control cells expressing YFP and CFP separately, yielding efficiencies ~0. ( e ) A versus sensor distance from channel mouth ( r sensor ), calculated with Neher-Stern equation (equation (1)), using parameters [13] , [60] D Ca =0.4 μm 2 ms −1 and k Bon =10 −3 μM −1 ms −1 for EGTA. Grey curves, plots with f values as labelled. Mapping A from ( b ) with r sensor from ( d ) yields f ~0.53 (black curve) and range (0.4-0.7, shading). ( f ) Schematic, idealized fenestrated Ca 2+ egress from inner channel mouth. Green cones, permissive radial diffusion paths from source (green dot), summing to f ~0.53. Target molecule (grey ball) within/near portal enjoys preferential signalling. Full size image The fusion of Ca V 2.2 channels to the genetically encoded Ca 2+ sensor TN–XL here furnishes a new tool for detecting submembranous Ca 2+ signals near these 'N-type' Ca 2+ channels ( Fig. 1b ). Our particular application concerns the nanodomain Ca 2+ transients accompanying individual channel openings and closings. These transients have eluded direct experimental comment, until the recent advent of TIRF microscopy to image single-channel activity [30] , [31] , and the availability of targetable chemical-fluorescent Ca 2+ indicators [38] . Here we demonstrate an alternative approach exploiting TIRF/patch–clamp electrophysiology and our Ca V 2.2/TN–XL fusion. This tactic yields a first empirical estimate of the amplitude of nanodomain Ca 2+ pulses ( Ca spike ). This parameter figures crucially in the Ca 2+ activation of co-localized channels and enzymes [2] , evoked release of nearby neurotransmitter vesicles [25] , and excitation–transcription coupling [8] , [9] . A limitation of the present study concerns the incomplete targeting of active Ca V 2.2/TN–XL channels to the surface membrane in the TIRF volume, necessitating approximate correction of static background fluorescence. The potential error in such correction renders our Ca spike determination as a coarse approximate estimate. Nonetheless, the approach taken will prove valuable as a means to improve channel trafficking arise, and GECI technology progresses. With this proviso, we consider other long-sought-after Ca 2+ channel signalling properties that could, in principle, be accessed with our strategy. First, we estimate the gain factor A , defined as the ratio of Ca spike to unitary current i fluxing through individual Ca 2+ channels [12] . As such, the magnitude of A is crucial for local Ca 2+ channel signalling to downstream nanodomain targets. Given knowledge of Ca spike , we could estimate A itself, so long as the i were known under the conditions of Ca spike determination ( Fig. 6 , with 10 mM Ca 2+ as the charge carrier). The single-channel data thus far ( Fig. 3c,d ) were obtained with 90 mM Ba 2+ to facilitate resolution of open probability; these data could not be utilized here. The relevant single-channel data for parameter A specification would entail several-fold smaller signals [25] , [52] . Nonetheless, despite signals near the limits of detection, we acquired well-resolved unitary currents under these conditions ( Fig. 7a ). These data yield i =0.085±0.003 pA ( n =5 patches) at 30 mV (as in Fig. 6 ), resembling values recorded in native Ca V 2.2 channels [25] . Combining i with our estimates of Ca spike (centre, ~60 μM; range, 45–80 μM), we obtain A , ~700 μM/pA ( Fig. 7b , shaded regions). Second, if the distance from the cytoplasmic mouth of the channel to the sensor ( r sensor ) were also known, near-field Ca 2+ sensing could comment powerfully on Ca 2+ diffusion within the nanodomain itself. We therefore gauge r sensor from FRET measured between the CFP of our Ca V 2.2/TN–XL fusion, and YFP fused to the base of the channel amino terminus ( Fig. 7c ). To eliminate crosstalk, YFP within TN–XL itself is replaced with the inert analogue amber [53] . FRET efficiency was thus determined [54] ( Fig. 7d ), yielding an estimated r sensor ~55 Å (Methods). With both parameter A and r sensor in hand, we scrutinize nanodomain Ca 2+ diffusion via classic point-source Ca 2+ diffusion, as given by a generalized Neher-Stern equation [13] , [16] where r sensor is the distance of the TN–XL sensor from the point source of Ca 2+ influx; D Ca is the diffusion coefficient of free Ca 2 ; F is Faraday's constant; k Bon is the on rate for Ca 2+ binding to EGTA; and B T is the internal EGTA concentration (10 mM). The parameter f , specifying the fraction of half-infinite space into which radial Ca 2+ diffusion occurs, has always been set at unity (Ca 2+ diffuses into a full half-infinite space), absent any evidence to the contrary. Intriguingly, our estimates of A and r sensor square poorly with the traditional view ( Fig. 7e , grey curve with f =1), but fit well with f ~0.53 (0.53×2 π steradians, solid curve). This outcome may represent an early functional indication of fenestrated Ca 2+ egress from the channel into cytoplasm ( Fig. 7f ), according with crystallographic structures of K channels [55] . Thus, nanodomain Ca 2+ diffusion could focus Ca 2+ through particular molecular geometries within the channel-signalling complex, raising the possibility of enhanced preferential signalling to target molecules near or within exit portals ( Fig. 7f , grey ball). Indeed, although previous studies elegantly suggest that distinctive unitary current amplitudes i render Ca V 2.2 channels favourable for triggering vesicle fusion [25] , it is also plausible that differing A and f values also factor into such optimization. The latter possibilities represent an intriguing, but nearly unexplored, realm of Ca 2+ biology. Although other interpretations are certainly viable, further empirical estimates of Ca spike , parameter A , and r sensor will likely aid in the dawning of this field of inquiry. Molecular biology Ca V 2. 2/TN–XL (Ca V 2.2 is of human origin (NM000718)) fusion construct was made by PCR, using fusion primers. Pfu polymerase (Strategene) was used for fidelity. To make Ca V 2.2/TN–XL, we first generated a Ca V 2.2 channel with the C-terminus truncated at the 2180th amino acid (without a stop codon), yielding Ca V 2.2Δ2180 stopless/XbaI in pcDNA3.1. This was made by cutting Ca V 2.2 with Xho I and Xba I, and replacing the resulting fragment with the PCR product amplified from Ca V 2.2 between the Xho I and 2180th amino-acid sites using forward primer 5′-CGCATCAGTTACAATGACATG-3′, and reverse primer 5′-CTGTCTAGAAGCACCAGATGTTGACAGCA-3′. Next, TN–XL was PCR-amplified with an Xba I site upstream of CFP (ATG removed) and a Nhe I/Spe I site downstream of the stop codon of circularly permuted Citrine. The forward and reverse primers used were 5′-CGGCCGCCACCTCTAGAGTGAGC-3′, and 5′-CAGACTAGTGCTAGCTTAGTCCTCGATGTTGTGGC-3′ respectively. Finally, the TN–XL PCR fragment was spliced into the Ca V 2.2Δ2180 stopless/XbaI construct at the Xba I site to give our Ca V 2.2/TN–XL construct. For the variant construct in Fig. 7c , the circularly permuted Citrine in TN–XL was replaced with circularly permuted amber [53] , and YFP fused to the amino terminus of Ca V 2.2 after removal of the first 81 amino acids [22] (nearly the entire amino terminus). Complete sequence analysis of regions subjected to PCR was performed. HEK293 cell culture and transfection HEK293 cells were cultured on No-1 25-mm glass cover slips (Bellco glass) in 10 cm plates. These slips were coated overnight with 0.01% (wt/v; diluted 1:5 in 0.1 M borate buffer) poly-d-lysine (Sigma), and washed with ddH 2 O on the day cells were seeded onto the slips. The poly-d-lysine coating facilitates proper whole-cell voltage control at the membrane/glass interface [56] , and also increases electrostatic attraction between the glass surface and cells, thus favouring cell attachment and optimal TIRF imaging. Cells were transiently transfected, using calcium-phosphate precipitation [54] , with Ca V 2.2/TN–XL, rat brain β 2a [54] , and rat brain α 2δ [54] (10 μg each). Ca V 2.2 and β 2a -CFP were substituted for Ca V 2.2/TN–XL and β 2a , respectively, in some experiments. Co-transfection of channels with a number of molecules did not appreciably improve channel trafficking in our system: PI3K and Akt/PKB [57] , ORL receptors [58] , and dominant-negative dynamin [59] . TN–XL and TN–XL-Ras sensors were transfected using FuGENE6 (Roche). Electrophysiology Whole-cell and single-channel current records were obtained at room temperature 1–3 d post-transfection, using patch–clamp amplifiers Axopatch 200B and Axopatch 200A (Axon Instruments), respectively. For whole-cell recordings, the cells were bathed in external solution containing (in mM): TEA-MeSO 3 , 140; HEPES (pH 7.4 with TEA-OH), 10; and CaCl 2 , 10; at 300 mOsm, adjusted with glucose. The internal solution contained (in mM): Cs-MeSO 3 , 114–135; CsCl, 5; EGTA, 1 or 10; MgCl 2 , 1; MgATP, 4; HEPES (pH 7.4 with CsOH), 10; and 295 mOsm with Cs-MeSO 3 . In some experiments, 10 μM Fluo 4FF and 2.5 μM Alexa 568 (Invitrogen, Molecular Probes) were included for ratiometric Ca 2+ determination. Electrodes were pulled from borosilicate glass capillaries (WPI MTW 150-F4) and had pipette resistances ranging from 1.5 to 2.5 MΩ before 75% series resistance compensation. Voltage pulses were applied at 90 s intervals. Currents were filtered at 5 kHz, and digitized at 25 kHz. Leak and capacitance transients subtracted by P/8 protocol. Data acquired and analysed with custom MATLAB scripts (Mathworks, Natick, MA, USA). Single-channel recordings were all conducted in the on-cell configuration. The bath contained (in mM): K Glutamate, 132; KCl, 5; NaCl, 5; MgCl 2 , 3; EGTA, 2; glucose, 10; and HEPES (pH 7.4 adjusted with KOH), 20 at 300 mOsm adjusted with glucose. This bath solution zeroed the membrane potential. The pipette solution contained, (in mM): BaCl 2 , 90; TEA-MeSO 3 , 20; HEPES (pH 7.4 adjusted with TEA-OH), 10 at 300 mOsm, adjusted with TEA-MeSO 3 . In some experiments, 10 mM CaCl 2 was substituted for BaCl 2 and TEA-MeSO 3 correspondingly increased. To minimize electrical noise, 5–20 MΩ patch pipettes were pulled from ultra-thick-walled (2 mm outer diameter, 1.16 mm inner diameter) borosilicate glass (BF200-116-10, Sutter Instruments), and coated with Sylgard. Seal resistance was ~80 GΩ. Voltage pulses applied at repetition intervals of 5–15 s; data sampled at 70 μsec intervals, and filtered at 2 kHz ( Fig. 3c,d ) or 700 Hz ( Fig. 7a ). TIRF microscopy On the day of experiments, the cover slips on which cells were cultured were mounted on a custom bath chamber for TIRF imaging. Fluorescence measurements of single cells were performed on a Nikon Eclipse TE2000U microscope, equipped with a Plan Apo 60× TIRF objective (NA 1.45 oil immersion). Nikon immersion oil, with nd=1.515 (23 °C) was used. For TN–XL imaging, CFP excitation was delivered by a 16-mW Melles Griot 56ICS 442-nm diode laser. For Fluo 4FF/Alexa 568 imaging, excitation was delivered by a 40-mW Melles Griot IMA100 argon laser featuring a 514-nm line. For TN–XL imaging, the optical path diagrammed in Supplementary Fig. S4 was used, as described below. A high-resolution CoolSNAP HQ CCD camera (Photometrics), driven by IPLab (Scanalytics) scientific imaging software, was used for cell orientation and verification under TIRF microscopy. Fast quantitative data, averaged across single cells, were instead acquired via photomultiplier tubes (PMTs), as follows. Single-cell fluorescent signals was selected by the image-plane pinhole in a D-104C dual-channel photometer (PTI), and sent to a dichroic mirror (510dclp) that divides the fluorescence emission signals into CFP and FRET signals. These two signals passed through their respective emitters (HQ485 per 30 m and HQ545 per 40 m, Chroma), before being captured by two Hamamatsu R1527 PMTs. Fluorescent signals were filtered at 2 kHz and sampled at 25 kHz, and reflect the activity of several thousand Ca V 2.2/TN–XL molecules. Shutter control, dark-current subtraction, and data acquisition were controlled by custom MATLAB programs. For Fluo 4FF/Alexa 568 imaging, the optical path was modified slightly. Single-cell fluorescence was isolated via the same pinhole and then sent to a dichroic mirror (545 dclp) that parsed signals into Fluo 4FF and Alexa 568 signals. These two signals passed through their respective emitters (545/40 nm bandpass and HQ580 nm lp, Chroma), before being captured by the same PMTs. The apparent K d for Fluo 4FF/Alexa 568 ratios under our recording conditions was 20 μM, as determined in live HEK293 cells dialysed with Ca 2+ dye and a series of calibrated [Ca 2+ ] internal solutions. Widefield FRET microscopy 3 3 -FRET efficiency determination, along with estimation of the ratio of donor to acceptor molecules, was performed within individual live HEK293 cells imaged through a image-plane pinhole according to CFP, FRET and YFP filter cubes [54] . Moreover, r sensor in Fig. 7d was estimated using a Forster distance of 49 Å (ref. 54 ). Immunoblots HEK293 cells expressing Ca V 2.2/TN–XL or TN–XL-Ras, were washed and collected with PBS, centrifuged and resuspended in lysis buffer (20 mM Tris–HCl [pH 7.5], 300 mM sucrose, 1 mM DTT and protease inhibitor cocktail (Roche)). Lysis was completed with freeze-thaw cycles and sonication. Membrane proteins were separated by initial centrifugation (16,000 g ×10 min at 4 °C), followed by solubilizing the resulting pellet in 1% Triton X-100. This solution was then subjected to centrifugation (16,000 g ×10 min at 4 °C), yielding membrane proteins in the supernatant. Membrane proteins were denatured (95 °C×1 min) on dilution with TGS buffer (Bio-Rad), and resolved by 5% SDS–PAGE with no CaCl 2 added to the gel. Proteins were transferred to nitrocellulose membranes (Bio-Rad) by cooled transfer (Tris/Glycine transfer buffer/pH 8.3×19 h). After blocking, membranes were sequentially incubated with rabbit polyclonal anti-GFP antibody (Abcam, 1:5,000 dilution, as directed by manufacturer) and HRP-conjugated secondary antibody (Sigma, 1:2400 dilution as recommended by manufacturer). Protein bands were visualized with enhanced chemiluminescence (Pierce ECL, Thermo Scientific). Data analysis and modelling Single-channel ramp data were analysed for Ca V 2.2/TN–XL. unitary current and open probability using custom MATLAB programs [10] . For the analysis, all patches contained 1 or 2 active channels. TIRF fluorescent signals from Ca V 2.2/TN–XL were modelled using custom MATLAB scripts, using approaches detailed in Supplementary Methods Generalization of the Neher-Stern equation (equation (1)), for f values other than unity, was accomplished by considering mass balance and substituting Q 1 / f for Q 1 in equation 6 of the original Stern paper [13] . How to cite this article: Tay, L. H. et al . Nanodomain Ca 2+ of Ca 2+ channels detected by a tethered genetically encoded Ca 2+ sensor. Nat. Commun. 3:778 doi: 10.1038/ncomms1777 (2012).